Offspring production with sperm grownin vitrofrom cryopreserved testis tissues With the increasing cure rate of paediatric cancers, infertility, as one of the adverse effects of treatments, has become an important concern for patients and their families. Since semen cryopreservation is applicable only for post-pubertal patients, alternative pre-pubertal measures are necessary. Here we demonstrate that testis tissue cryopreservation is a realistic measure for preserving the fertility of an individual. Testis tissues of neonatal mice were cryopreserved either by slow freezing or by vitrification. After thawing, they were cultured on agarose gel and showed spermatogenesis up to sperm formation. Microinsemination was performed with round spermatids and sperm, leading to eight offspring in total. They grew healthily and produced progeny upon natural mating between them. This strategy, the cryopreservation of testis tissues followed by in vitro spermatogenesis, is promising to preserve the fertility of male paediatric cancer patients in the future. Among all cancer patients, the proportion of those under 20 years old is ~1% (ref. 1 ). These cancers include leukaemia, Hodgkin’s lymphoma and testis cancer, which are aggressive and progress rapidly. Recent advances of treatment modalities, however, have significantly increased the survival rate of such juvenile patients up to 70–90% (ref. 1 ). It was reported that about one in 640 adults aged from 20 to 39 years old were survivors of paediatric cancers in a nationwide study in the United States of America [2] . Thus, infertility caused by cancer treatments has become a serious concern for patients and their families. Although semen cryopreservation, as a countermeasure, is widely practised and useful, it is not applicable to patients before puberty. Cryopreservation of testis tissues has been proposed as a measure to preserve fertility in boys planned to undergo cytoablative cancer treatments [3] , [4] . There have been several reports of animal experiments based on such an idea [3] , [5] , [6] , [7] . These reports demonstrated the efficacy of testis tissue cryopreservation as a means to preserve fertility. However, all reports depended on grafting or transplantation methods to obtain sperm from frozen samples. Such procedures are invasive for patients and, more importantly, carry the risk of re-introducing malignant cells, especially in leukaemia patients [8] , [9] . Xeno-grafting is a possible alternative, but it is associated with other concerns, beside its efficiency, such as whether gametes grown in an animal body carry fragments of DNA or viruses of animal origin [10] . Recently, we revisited a classical organ culture method, the air–liquid interphase method, and successfully modified it to induce complete spermatogenesis of mice in vitro [11] . In this previous work, we found that spermatogenesis could be induced even in frozen tissues. To confirm this preliminary result and test the competency of the resulting sperm, we refined the cryopreservation method and performed microinsemination experiments. The resulting offspring were healthy and reproductively competent when matured, demonstrating that this measure could be clinically applicable in the future. Optimization of freezing method First, we examined two freezing methods and several cryoprotectants by evaluating the spermatogenic potential of tissues following different methods of cryopreservation. The two freezing methods were slow freezing and vitrification, the latter of which is now widely used in clinical settings for oocytes, embryos and ovarian tissues [12] , [13] , [14] . As cryoprotectants, dimethylsulphoxide (DMSO), propanediol (PROH) and Cell Banker 1 (CB) were used for slow freezing and Stem Cell Keep (SCK) was used for vitrification. Testis tissues at 4.5 days post partum (d.p.p.) from Gsg2 -GFP transgenic mice ( Gsg2 -Tg), whose spermatogenic cells express green fluorescent protein (GFP) from the late meiotic stage onward [15] , were cryopreserved. After being preserved in liquid nitrogen for 7 or 8 days, they were thawed and cultured on agarose gel to promote spermatogenesis [11] . The progression of spermatogenesis was evaluated by the level of GFP expression [11] in each tissue. Experiments were repeated five times. The GFP expression levels were always highest in DMSO and SCK groups, and even comparable to unfrozen control samples ( Fig. 1a ). This favourable expression of Gsg2 -GFP reflects the progression of spermatogenesis. For example, in 5.5 d.p.p. mice, after being vitrified and cryopreserved in liquid nitrogen for 202 days, the tissues expressed GFP from culture day 24 until day 46 ( Fig. 1b ). This sample was processed for immunostaining, which demonstrated the presence of spermatocytes in the pachytene stage based on the positive signal of synaptonemal complex protein 1 (SYCP1) ( Fig. 1c ). Many round spermatids were positive for peanut agglutinin along their acrosomal contour ( Fig. 1c ). Histological observation of a sample that originated from 4.5 d.p.p., preserved for 187 days, and cultured for 43 days revealed that elongating spermatids were produced sporadically along with round spermatids in the seminiferous tubules ( Fig. 1d ). Sperm were confirmed in dissociated samples ( Fig. 1e ). Among the 30 cultured tissues that were chosen for dissociation because of their extensive expression of Gsg2 -GFP or Acr -GFP, we found sperm in 17 tissues. Among them, more than 100 sperm were found in each of 7 tissues and more than 10 sperm in each of 6 tissues ( Fig. 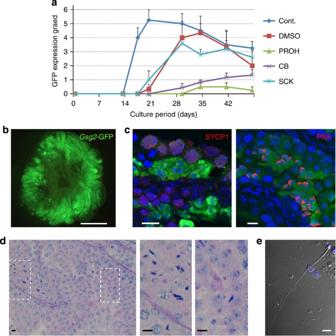Figure 1: Effect of freezing methods and cryoprotectants onin vitrospermatogenesis. (a) Time course ofGsg2-GFP expression grades of testis tissues treated with four cryopreservation methods and the non-frozen control represented by the average and SEM. The numbers of testis tissues examined were four (control, Cont.), three (DMSO), four (PROH), six (CB) and five (SCK). (b) GFP expression image of testis tissue, from 5.5 d.p.p.Gsg2-Tg mice, cryopreserved with SCK for 202 days and cultured for 46 days. Scale bar, 1 mm. (c) The same sample was processed for immunostaining with SYCP1 (red, left) indicating meiotic cells, and peanut agglutinin (red, right) indicating round spermatids. The tissues were also stained with GFP (green) and counterstained with Hoechst (blue). Scale bars, 10 μm. (d) Histologic view with Periodic acid-Schiff staining of culture tissues, demonstrating round and elongating spermatids. The tissue originates from 4.5 d.p.p.Gsg2-GFP Tg mice testis cryopreserved with SCK for 187 days and cultured for 42 days. The dotted rectangular areas are enlarged on the right. Scale bars, 10 μm. (e) Sperm were confirmed in dissociated samples, from 2.5 d.p.p.Gsg2-GFP Tg mice, cryopreserved with SCK for 145 days and cultured for 42 days. Stained with Hoechst. Scale bar, 10 μm. 2 and Table 1 ). This sperm retrieval rate is comparable to that using fresh tissues samples; the sperm retrieval rate was ~50% in tissues expressing Acr - or Gsg2 -GFP in over 30% of the tissue area corresponding to grade 3 or higher. Figure 1: Effect of freezing methods and cryoprotectants on in vitro spermatogenesis. ( a ) Time course of Gsg2 -GFP expression grades of testis tissues treated with four cryopreservation methods and the non-frozen control represented by the average and SEM. The numbers of testis tissues examined were four (control, Cont. ), three (DMSO), four (PROH), six (CB) and five (SCK). ( b ) GFP expression image of testis tissue, from 5.5 d.p.p. Gsg2 -Tg mice, cryopreserved with SCK for 202 days and cultured for 46 days. Scale bar, 1 mm. ( c ) The same sample was processed for immunostaining with SYCP1 (red, left) indicating meiotic cells, and peanut agglutinin (red, right) indicating round spermatids. The tissues were also stained with GFP (green) and counterstained with Hoechst (blue). Scale bars, 10 μm. ( d ) Histologic view with Periodic acid-Schiff staining of culture tissues, demonstrating round and elongating spermatids. The tissue originates from 4.5 d.p.p. Gsg2 -GFP Tg mice testis cryopreserved with SCK for 187 days and cultured for 42 days. The dotted rectangular areas are enlarged on the right. Scale bars, 10 μm. ( e ) Sperm were confirmed in dissociated samples, from 2.5 d.p.p. Gsg2 -GFP Tg mice, cryopreserved with SCK for 145 days and cultured for 42 days. Stained with Hoechst. Scale bar, 10 μm. 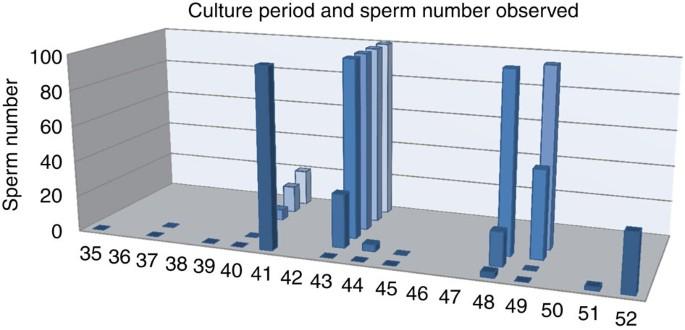Figure 2: Numbers of sperm observed in each dissociated testis tissue at each time point. Cultured tissues were mechanically dissociated for examination. Sperms were identified from corresponding donor age of 40-day onward. Full size image Figure 2: Numbers of sperm observed in each dissociated testis tissue at each time point. Cultured tissues were mechanically dissociated for examination. Sperms were identified from corresponding donor age of 40-day onward. Full size image Table 1 Culture period and sperm number observed. Full size table Fertility of sperm and spermatids obtained from cryopreserved tissues We performed three sets of microinsemination experiment with tissues cryopreserved with CB or SCK ( Tables 2 and 3 ). In the first experiment (insemination exp. 1), neonatal testis tissues of Acrosin -GFP Tg ( Acr -Tg) or Gsg2 -Tg, aged 1.5–3.5 d.p.p., which were cryopreserved with CB for 18–143 days, were thawed and cultured. 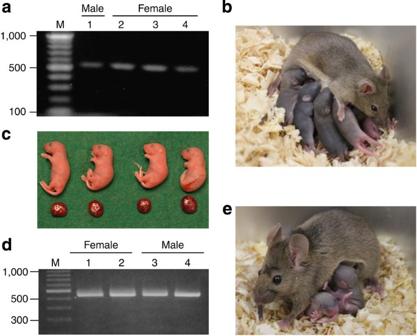Figure 3: Results of microinsemination experiments. (a) Four offspring were produced with ROSI using round spermatids harvested from cryopreserved tissue with the cryoprotectant CB. Genomic DNA analysis confirmed their origin asGsg2-GFP Tg. The amplified enhanced GFP (EGFP)–DNA size is 538 bp. (b) The offspring grew healthily and produced the next generation by sibling mating. (c) Four offspring were produced by ICSI using sperm derived from tissues vitrified with SCK. (d) Tail-tip DNA was subjected to PCR analysis, showing that all four pups were positive for GFP. Amplified EGFP–DNA was 538 bp. (e) The offspring grew healthily and produced the next generation by mating between progenies. Among the 231 tissue pieces cultured, we selected 21 based on the expression level of GFP at around 43 days of culture to harvest haploid cells for microinsemination ( Table 3 ). Among these 21 tissues, one tissue contained haploid cells and we obtained 17 round spermatids and 8 sperm, which were used for microinsemination. Finally, four progeny were produced following round spermatid injection (ROSI; Tables 2 and 3 ). Genomic PCR of these four mice confirmed the presence of the GFP gene ( Fig. 3a ). Natural mating between siblings produced the next generation ( Fig. 3b ). In the second experiment (insemination exp. 2), testis tissues were cryopreserved by the vitrification method with SCK ( Table 3 ). Eleven tissues were chosen from samples of seven independent culture experiments. In five tissues, we found seven sperm and 78 round spermatids in total, which were used for microinsemination. Although eight implantations were observed, no offspring were obtained ( Tables 2 and 3 ). In the third experiment (insemination exp. 3), 20 tissues were selected from samples of eight independent culture experiments to obtain sperm ( Table 3 ). In eight tissues, originating from two experiments, 68 sperm were obtained for microinsemination. Among the 68 fertilized eggs, 42 eggs underwent cell division and were transferred to oviducts of females. Eighteen implantations were observed, and four offspring were obtained ( Fig. 3c and Table 2 ). These four mice carried the GFP gene, indicating their origin from cultured tissues, and grew healthily ( Fig. 3d ). They also produced the next generation by natural mating between progeny ( Fig. 3e ). On the other hand, ROSI with 58 round spermatids was unsuccessful in this set of experiments on microinsemination ( Tables 2 and 3 ). To test if there is any methylation abnormality in the offspring, 11 germline differentially methylated regions (DMRs; H19 , IG, Rasgrf1, Igfr2r , Lit1 , Meg1 , Peg1 , Peg3 , Peg10 , Peg13 and Snrpn ) were examined with the Combined Bisulfite Restriction Analysis (COBRA) method. The DNA methylation levels at DMRs in both ROSI-derived and intracytoplasmic sperm injection (ICSI)-derived animals were practically equal to those of the control at all sites examined ( Supplementary Fig. 1 ). Table 2 Summary of microinsemination experiments. Full size table Table 3 Cryopreservation and organ culture experiments. Full size table Figure 3: Results of microinsemination experiments. ( a ) Four offspring were produced with ROSI using round spermatids harvested from cryopreserved tissue with the cryoprotectant CB. Genomic DNA analysis confirmed their origin as Gsg2 -GFP Tg. The amplified enhanced GFP (EGFP)–DNA size is 538 bp. ( b ) The offspring grew healthily and produced the next generation by sibling mating. ( c ) Four offspring were produced by ICSI using sperm derived from tissues vitrified with SCK. ( d ) Tail-tip DNA was subjected to PCR analysis, showing that all four pups were positive for GFP. Amplified EGFP–DNA was 538 bp. ( e ) The offspring grew healthily and produced the next generation by mating between progenies. Full size image In this study, we found that methods of cryopreservation along with the choice of cryoprotectant affected the condition of preserved tissues, leading to differences in spermatogenic efficiency during the following cultivation period. Among the methods we tested, tissues undergoing vitrification with SCK as a cryoprotectant showed spermatogenesis comparable to that of unfrozen control experiments. This may indicate that the cryopreservation method is not as critical as the culture conditions, such as the culture medium or temperature, regarding the outcome of sperm production. In other words, improvement of the culture conditions is more important to increase the rate of harvesting sperm from cryopreserved tissues. In fact, our organ culture system is far from ideal and has much room for improvement. In particular, our culture medium, being useful for mouse tissue, does not work with rat tissue. Thus, optimization of the medium formula may be necessary for each animal species. Another drawback of our culture system is that it depends on Knockout Serum Replacement (KSR) or AlbuMAX, whose components have not been fully revealed, and this may impede improvement of the culture medium. In addition, as both products were produced from bovine serum, they would contain xeno-bioproducts, thereby limiting their use in human clinics. Therefore, a system is needed with chemically defined medium conditions. These limitations and challenges, however, when resolved, will guarantee a deeper understanding of the mechanism of spermatogenesis in many species, including humans. Another concern with this strategy is the fidelity and safety of the sperm produced from cryopreserved tissue under in vitro conditions. We addressed this issue by checking the status of imprinting genes of the offspring, because epigenetic changes in imprinting genes are the most likely abnormalities induced by embryo culture and artificial reproductive manipulations [16] , [17] . The data showed that all 11 DMRs examined showed an almost normal state of methylation. This result, however, is not sufficient to guarantee the normality of the sperm’s imprinting gene status. The quality evaluation of sperm is critically important for application in future clinical practice. Thus, the systemic examination of the epigenetic status of such sperm produced in vitro , with or without cryopreservation, is warranted. On the other hand, there have been several reports on germ cell production from pluripotent stem cells under culture conditions [18] , [19] . Such technology would be a last resort for patients who have totally lost germ-lineage cells and had been unable to preserve their gametes or gonadal tissues before the loss. However, the safety and fidelity of those germ cells differentiated in vitro from somatic cells should be examined properly before any clinical application. Organ culture of testis tissues for spermatogenesis seems to be more natural, because the microenvironmental condition for germ cells is close to that in vivo . Although they may not be easy and require further investigation, organ culture methods for the spermatogenesis of other animals including humans are expected to be successful in the future. When this goal is realized, testis tissue cryopreservation will become a practical means to preserve the reproductive capacity of pre-pubertal male cancer patients. The present data support developing this strategy for future clinical application. Mice and treatments Gsg2 -GFP transgenic mice [15] and Acr -GFP transgenic mice [20] , [21] (genetic background: ICR, C57BL/6 and their mixture) were mated with female mice of ICR, C57BL/6, or their hybrid descendants to produce pups. Immature testis tissues were obtained from mice at 0.5–5.5 d.p.p. Mice were killed by decapitation, and then the testes were excised and rinsed in αMEM (Invitrogen, cat. no. 12000-022) +10% KSR; Invitrogen, cat. no. 10828-028) on ice. The tunica albuginea was removed and testes were divided into 2–3 pieces with forceps. All of the animal experiments conformed to the Guide for Care and Use of Laboratory Animals and were approved by the Institutional Committee of Laboratory Animal Experimentation (Research Institute for Yokohama City University, Yokohama, Japan). Cryopreservation and thawing Tissue pieces of ~1 mm 3 were cryopreserved by either conventional slow freezing or vitrification. For slow freezing, three cryoprotectant solutions were used: first solution: αMEM+10% KSR containing 0.05 M of sucrose and 1.5 M of DMSO solution, second solution: αMEM+10% KSR containing 0.05 M of sucrose and 1.5 M of PROH solution, and third solution: Cell Banker 1 (Juji Field, Inc., Tokyo, Japan). For vitrification, Stem Cell Keep (Bioverde, Kyoto, Japan) was used as a cryoprotectant. Two to six pieces of tissue were transferred into a Cryogenic Vial (Sumitomo Bakelite, Tokyo, Japan) containing 200 μl of cryoprotectant. In the case of DMSO or PROH solution, the tissues were put into a Cryogenic Vial (1.5 ml) containing 200 μl of each solution for 30 min at 4 °C. The cryovials containing tissues were then stored in a Bicell biofreezing vessel (Nihon Freezer Co., Ltd, Tokyo, Japan) and placed in a deep freezer at −80 °C overnight. Tissue samples in the Bicell device were cooled down at a rate of ~1 °C per min in a deep freezer until reaching −80 °C. Then, the vials were plunged into liquid nitrogen. For thawing, the vials were incubated at 37 °C in a water bath for ~2 min. The contents were emptied immediately into a dish that contained αMEM+10% KSR with sucrose (0.05 M) and DMSO (1.0 M) or PROH (1.0 M). After 5 min of rinsing, tissues were transferred into another medium of αMEM+10% KSR with sucrose (0.05 M) and 0.5 M of DMSO or PROH for 5 min rinsing. Then, tissues were rinsed in a dish that contained αMEM+10% KSR with sucrose (0.05 M) for 5 min. Finally, the tissues were rinsed in αMEM+10% KSR for 5 min and transferred to the agarose gel. In the case of CB, tissues were put in a cryogenic vial containing 200 μl of CB solution and held at 4 °C for 30 min. The vials were then simply placed in a deep freezer overnight and transferred into liquid nitrogen. For thawing, the vials were incubated at 37 °C and transferred to 1 ml of αMEM+10% KSR for rinsing, followed by three changes of the new medium before culturing. In the case of vitrification, fragments of testis tissue were put in cryogenic vials containing 200 μl of SCK for submerging at room temperature for 2 min. The vials were then plunged into liquid nitrogen. For thawing, cryovials taken out of the liquid nitrogen were quickly opened and αMEM+10% KSR pre-warmed at 37 °C was added. The tissue pieces were then transferred in αMEM+10% KSR for 5 min of rinsing at room temperature with three changes for new medium. Culture method Agarose gel of 1.5% (w/v), as a stand for tissues placement, was prepared. They were submerged in the culture medium, αMEM +10% KSR or αMEM with AlbuMAX (40 mg ml −1 ; Invitrogen), for a quarter to 1 day before use. Thawed tissue fragments were transferred to the flat surface of agarose gel that was half-soaked in the medium. Each gel was loaded with 1–3 tissue fragments. Medium change was performed once a week. The culture incubator was supplied with 5% carbon dioxide in air and maintained at 34 °C. The protocol was reported previously in detail [22] . Gross and histological examination Cultured tissues were occasionally observed under a stereomicroscope to evaluate the progress of spermatogenesis based on the extent of the GFP-expressing area, which corresponds with the area showing spermatogenesis in the mid-meiotic phase or beyond. Under observation with a stereomicroscope equipped with an excitation light for GFP (Olympus SZX12; Olympus, Tokyo, Japan), the area showing GFP expression was roughly measured and classified into six grades: ~10, ~30, ~50, ~70, ~90 and ~100% (ref. 11 ). For histological examination, the specimens were fixed with Bouin’s fixative and embedded in paraffin. One section showing the largest cut surface was made for each specimen and stained with haematoxylin and eosin or Periodic acid-Schiff. To search for spermatids and sperm, cultured tissues were mechanically dissociated using needles to release cells into the phosphate-buffered saline (PBS). The cell suspension was stained with Hoechst 33342 dye and observed with a microscope under GFP excitation light. Immunohistochemistry Tissues were fixed with 4% paraformaldehyde in PBS at 4 °C overnight. They were cryoembedded in OCT compound (Sakura Finetechnical, Tokyo, Japan) and cut into 7-μm-thick sections. Incubation with primary antibodies was performed overnight at 4 °C, followed by rinsing twice with PBS containing Triton X-100 (0.2%), and then secondary antibodies were applied for 1 h at room temperature. Nuclei were counterstained with Hoechst 33342 dye. Specimens were observed with a confocal laser microscope (FV-1000D; Olympus). The following were used as primary antibodies: rat anti-GFP antibody (1:1,000, Nakalai Tesque, Inc., Kyoto, Japan), rabbit anti-SYCP1 antibody (1:600, Novus Biologicals) and rabbit anti-peanut agglutinin antibody (1:400, Novus Biologicals). The secondary antibodies used were goat anti-rabbit IgG and goat anti-rat IgG, conjugated with Alexa 488 or Alexa 555 (1:200; Molecular Probes). Microinsemination The cultured testis tissues were dissected out under a stereomicroscope. Round spermatids or spermatozoa were collected and injected into the ooplasm of mature wild-type oocytes of B6D2F1 using a Piezo-driven micromanipulator [23] . For fertilization with round spermatids, oocytes were then activated by treatment with SrCl 2 in the presence of cytochalasin B to resume meiosis. After the formation of two female pronuclei, one was removed with a micropipette [23] . Fertilized oocytes were cultured for 24 h, and two-cell embryos were transferred into the oviducts of pseudopregnant ICR females. Live fetuses retrieved on day 19.5 were raised by lactating foster ICR dams. PCR analysis Genomic DNA was extracted from the mouse tail with a DNeasy Tissue kit (Qiagen). The DNA samples (~10 ng) were added to a 20-μl reaction mixture containing 0.25 μM of each enhanced GFP-specific primer and Premix ExTaq (Takara Bio). Enhanced GFP-specific primers were 5′-TACGGCAAGCTGACCCTGAA-3′ and 5′-TGTGATCGCGCTTCTCGTTG-3′. The reaction profile was: four cycles of denaturation at 98 °C for 10 s, annealing at 65 °C for 30 s and extension at 72 °C for 30 s, and then 31 cycles of denaturation at 98 °C for 10 s, annealing at 60 °C for 30 s and extension at 72 °C for 30 s. Combined bisulphite restriction analysis One microgram of genomic DNA was bisulphite-treated and purified using the EpiTect Bisulfite Kit (Qiagen). PCR amplification for COBRA assays for eleven imprinted, DMRs ( Supplementary Table 1 ) was performed in a total volume of 20 μl containing 20 ng of bisulphite-converted DNA, 20 pmol of each primer, dNTPs (2.5 mM each), 1.5 U of ExTaq HS (Takara) and supplied buffer. The standard thermal cycling conditions used were: initial denaturation at 94 °C for 5 min, followed by 35 cycles of denaturation at 94 °C for 30 s, annealing for 30 s and extension at 72 °C for 30 s (the annealing temperature for each primer pair is listed in Supplementary Table 1 ). The PCR products were purified using the Illustra GFX 96 PCR purification kit (GE Healthcare). One quarter of the purified PCR products were digested with 6 U of a restriction enzyme ( Supplementary Table 1 ) in a 15-μl scale reaction for 2 h. One μL was electrophoresed using the MultiNA Microchip Electrophoresis System and DNA-500 reagent kit (Shimadzu, Japan). The methylation rate for each sample was calculated as described previously [24] . How to cite this article: Yokonishi, T. et al. Offspring production with sperm grown in vitro from cryopreserved testis tissues. Nat. Commun. 5:4320 doi: 10.1038/ncomms5320 (2014).